Beclin 1 restrains tumorigenesis through Mcl-1 destabilization in an autophagy-independent reciprocal manner Mcl-1 is a unique Bcl-2 family member that plays crucial roles in apoptosis. Apoptosis-unrelated functions of Mcl-1 are however emerging, further justifying its tight regulation. Here we unravel a novel mechanism of Mcl-1 regulation mediated by the haplo-insufficient tumour suppressor Beclin 1. Beclin 1 negatively modulates Mcl-1 stability in a reciprocal manner whereby depletion of one leads to the stabilization of the other. This co-regulation is independent of autophagy and of their physical interaction. Both Beclin 1 and Mcl-1 are deubiquitinated and thus stabilized by binding to a common deubiquitinase, USP9X. Beclin 1 and Mcl-1 negatively modulate the proteasomal degradation of each other through competitive displacement of USP9X. The analysis of patient-derived melanoma cells and tissue samples shows that the levels of Beclin 1 decrease, while Mcl-1 levels subsequently increase during melanoma progression in a significant inter-dependent manner. The identified inverse co-regulation of Beclin 1 and Mcl-1 represents a mechanism of functional counteraction in cancer. Several types of tumours express abnormally high levels of Mcl-1 and numerous reports have established a direct link between elevated levels of Mcl-1 and tumorigenesis, drug resistance and relapse in those tumours [1] , [2] , [3] , [4] , [5] , [6] , [7] . Mcl-1 plays a key role in the regulation of apoptosis and its tumour-promoting properties have been largely attributed to its anti-apoptotic functions. However, emerging reports now suggest that Mcl-1 is implicated in other cellular processes that may contribute to its tumorigenic potential. Recently, Mcl-1 has been implicated in the regulation of mitochondrial bioenergetics and morphogenesis [8] , chemotherapy-induced senescence [9] , starvation and Ras oncogene-induced autophagy [10] , [11] , suggesting that its contribution to tumorigenesis may go beyond evading apoptosis. Targeting Mcl-1 is emerging as a potential therapeutic strategy [12] , [13] , [14] , [15] , [16] and therefore a deeper understanding of the mechanisms controlling Mcl-1 levels and function is of paramount importance. In comparison with other anti-apoptotic members of the Bcl-2 family, Mcl-1 exhibits some unique features including its tight regulation by complex mechanisms at the multiple levels of expression, translation and stability [17] . Beclin 1 is a haplo-insufficient tumour suppressor that is frequently deleted or downregulated in several types of tumours [18] , [19] , [20] , [21] . Enhanced expression of Beclin 1 is associated with inhibition of cellular proliferation and diminished in vitro clonogenic survival [11] and xenograft tumour growth [19] . Owing to its central role in autophagy, the tumour suppressor function of Beclin 1 has been initially associated with autophagy. However, it is not clear whether autophagy solely accounts for Beclin 1 tumour suppression capacity. Increasing evidence suggests that Beclin 1 may be involved in other processes that contribute to its tumour-restraining potential [22] , [23] . In the current study, we identify a novel mechanism of regulation of Mcl-1 mediated by the haplo-insufficient tumour suppressor Beclin 1 that at the same time acts as a mechanism of regulation of Beclin 1 itself in an inverse reciprocal manner. On the basis of our results, we propose that this reciprocal mechanism contributes to the opposite roles the two proteins play in the process of tumorigenesis. The ability of Beclin 1 to modulate Mcl-1 levels represents an autophagy-independent function of Beclin 1 that could account for an important part of its tumour-restraining capacity. Beclin 1 and Mcl-1 are reciprocally co-regulated Considering the emerging role of Mcl-1 in mediating starvation-induced autophagy [10] , [11] , [24] , we first assessed the contribution of endogenous Mcl-1 to the regulation of basal, housekeeping autophagy. Protein levels of Mcl-1, Bcl-2 or Bcl-xL were depleted by transiently transfecting 293T cells with two different siRNAs against each protein or a control siRNA against Luciferase. Depletion of endogenous Mcl-1 but not of Bcl-2 or Bcl-xL was sufficient to induce basal autophagy in cells cultured under nutrient-rich conditions as assessed by conversion of LC3I to II and decrease in p62 levels ( Fig. 1a ). Importantly, the induction of autophagy in response to Mcl-1 depletion was associated with a marked increase in the levels of Beclin 1 protein, not observed on depletion of Bcl-2 or Bcl-xL ( Fig. 1a ). The tight correlation between decrease in Mcl-1 and increase in Beclin 1 levels was further confirmed by transfecting 293T cells with a doxycycline-inducible shRNA construct targeted against Mcl-1. Cells were then either left untreated or treated with doxycycline for 1, 3 or 5 days. On doxycycline treatment, Mcl-1 levels gradually decreased, which was concomitant with proportional increase in the levels of Beclin 1 protein. In the same settings, the levels of other autophagy regulators, Atg5 and Atg7, remained unchanged, suggesting a specific counter regulation between Mcl-1 and Beclin 1 ( Fig. 1b ). To further explore these findings, Mcl-1 was pharmacologically depleted in 293T cells taking advantage of two kinase inhibitors known to affect Mcl-1 protein levels [17] . Treatment of 293T cells with either roscovitine or sorafenib, which block Mcl-1 transcription and translation, respectively, led to decrease in Mcl-1 and concomitant increase in Beclin 1 levels. The BH3 mimetic ABT 737 that does not target Mcl-1 failed to exert a similar effect, confirming the specificity of Beclin 1 modulation by Mcl-1 ( Fig. 1c ). 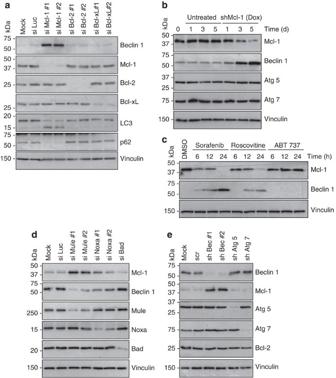Figure 1: Inverse correlation between Mcl-1 and Beclin 1 levels. (a) Assessment of autophagy markers in 293T cells transfected with the indicated siRNAs and grown in nutrient-rich medium. (b) Mcl-1 knockdown in 293T cells transfected with tetracycline-inducible shRNA against Mcl-1 and either treated with Doxycycline (100 ng ml−1) or left untreated for the indicated time points. (c) Pharmacological depletion of Mcl-1 in 293T cells treated with sorafenib (10 μM), roscovitine (25 μM) or ABT 737 (1 μM) as control for the indicated time points. (d) Stabilization of endogenous Mcl-1 and concurrent decrease in Beclin 1 in 293T cells transfected with the indicated siRNAs. (e) Mcl-1 upregulation upon Beclin 1 knockdown in 293T cells transfected with the indicated shRNAs. Figure 1: Inverse correlation between Mcl-1 and Beclin 1 levels. ( a ) Assessment of autophagy markers in 293T cells transfected with the indicated siRNAs and grown in nutrient-rich medium. ( b ) Mcl-1 knockdown in 293T cells transfected with tetracycline-inducible shRNA against Mcl-1 and either treated with Doxycycline (100 ng ml −1 ) or left untreated for the indicated time points. ( c ) Pharmacological depletion of Mcl-1 in 293T cells treated with sorafenib (10 μM), roscovitine (25 μM) or ABT 737 (1 μM) as control for the indicated time points. ( d ) Stabilization of endogenous Mcl-1 and concurrent decrease in Beclin 1 in 293T cells transfected with the indicated siRNAs. ( e ) Mcl-1 upregulation upon Beclin 1 knockdown in 293T cells transfected with the indicated shRNAs. Full size image Thus, RNAi-mediated or pharmacological depletion of Mcl-1 results in Beclin 1 upregulation. To further explore this inverse correlation between Mcl-1 and Beclin 1 levels, we sought to examine whether elevation of Mcl-1 levels may conversely lead to a decline in that of Beclin 1. Mcl-1 protein levels are controlled by proteasomal degradation as a consequence of ubiquitination by several E3 ligases including Mule [25] . It has also been reported that binding to the BH3-only protein Noxa targets Mcl-1 for proteasomal degradation [26] . To study the effect of elevation of endogenous Mcl-1 level on Beclin 1, 293T cells were transfected with two different siRNAs raised against either Mule or Noxa to stabilize Mcl-1. Depletion of Mule or Noxa led to varying magnitudes of increase in Mcl-1 levels depending on the efficiency of the knockdown, as shown in Fig. 1d . This increase in Mcl-1 was associated with a tightly corresponding decrease in Beclin 1 levels in each case. As a control, knocking down the BH3-only protein Bad, which had no effect on Mcl-1 levels, did not modulate Beclin 1 levels to any extent ( Fig. 1d ). Strikingly, when Beclin 1 protein levels were extinguished using two different shRNAs, Mcl-1 levels markedly increased indicating that the modulation between Mcl-1 and Beclin 1 is reciprocal. The extinction of other autophagy regulators such as Atg5 or Atg7, which act in the autophagy pathway downstream of Beclin 1, did not have any consequences on Mcl-1 levels ( Fig. 1e ) further confirming the specificity of Beclin 1/Mcl-1 interdependency and suggesting that this co-regulation is independent of the autophagy regulatory functions of Beclin 1. The same Beclin 1/Mcl-1 interdependency was also observed when we performed similar experiments in HeLa cells, suggesting that these observations are not limited to 293T cells ( Supplementary Fig. 1 ). Consistent with the observation that Beclin 1 can impact the stability of some of its interacting proteins, we also observed that ablation of Mcl-1 led to increase in UVRAG and Atg14 levels ( Supplementary Fig. 2 ). In conclusion, the data presented above indicate that Mcl-1 and Beclin 1 are co-regulated in a negative reciprocal manner whereby depletion of one leads to the upregulation of the other. Mcl-1 and Beclin 1 reciprocally modulate their ubiquitination To gain insight into the mechanism of reciprocal regulation between Mcl-1 and Beclin 1, we initially examined the expression of MCL1 and BECN1 genes in 293T cells depleted of either Beclin 1 or Mcl-1, respectively. No detectable changes in BECN1 gene expression was observed in cells transfected with two different siRNAs raised against Mcl-1 compared with control cells transfected with siRNA against Luciferase as shown by real-time qPCR ( Fig. 2a ). Similarly, when Beclin 1 levels were extinguished by two different shRNAs specific for the Beclin 1 transcript, no detectable changes in MCL1 gene expression were observed ( Fig. 2b ). 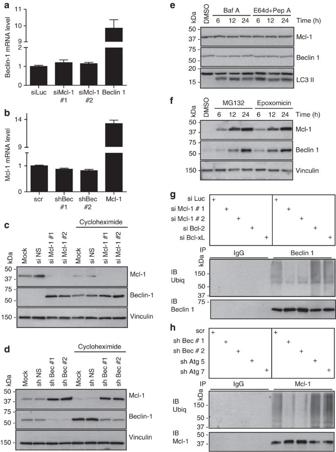Figure 2: Reciprocal regulation between Mcl-1 and Beclin 1 protein stability and ubiquitination. Beclin 1 (a) and Mcl-1 (b) mRNA levels in 293T cells transfected with the indicated siRNAs/shRNAs. Results are representative of at least three independent experiments. Error bars represent s.e.m. (c,d) Beclin 1 and Mcl-1 protein levels in 293T cells transfected with the indicated siRNAs/shRNAs and treated with or without cycloheximide (20 μg ml−1) for 6 h. (e,f) Mcl-1 and Beclin 1 protein levels in 293T cells treated with the inhibitors of either the lysosomal degradation pathway (100 nM Bafilomycin A, 10 μg/ml E64d+Pep) or the proteasome (2.5 μM MG132, 25 nM Epoximicin) for the indicated time points. (g,h) Beclin 1 or Mcl-1 were immunoprecipitated from 293T cells transfected with the indicated siRNAs/shRNAs and assessed for their ubiquitination levels. Figure 2: Reciprocal regulation between Mcl-1 and Beclin 1 protein stability and ubiquitination. Beclin 1 ( a ) and Mcl-1 ( b ) mRNA levels in 293T cells transfected with the indicated siRNAs/shRNAs. Results are representative of at least three independent experiments. Error bars represent s.e.m. ( c , d ) Beclin 1 and Mcl-1 protein levels in 293T cells transfected with the indicated siRNAs/shRNAs and treated with or without cycloheximide (20 μg ml −1 ) for 6 h. ( e , f ) Mcl-1 and Beclin 1 protein levels in 293T cells treated with the inhibitors of either the lysosomal degradation pathway (100 nM Bafilomycin A, 10 μg/ml E64d+Pep) or the proteasome (2.5 μM MG132, 25 nM Epoximicin) for the indicated time points. ( g , h ) Beclin 1 or Mcl-1 were immunoprecipitated from 293T cells transfected with the indicated siRNAs/shRNAs and assessed for their ubiquitination levels. Full size image We next investigated whether mRNA translation and protein biosynthesis play a role in the Beclin 1/Mcl-1 co-regulation. 293T cells were transfected with siRNAs targeted against Mcl-1 or Beclin 1 as described above and then treated with or without the protein translation inhibitor cycloheximide. As shown in Fig. 2c,d , inhibition of de novo protein synthesis by cycloheximide failed to modulate the increase in protein levels to any significant extent as compared with untreated cells, ruling out a role for protein translation. Taken together, these data demonstrate that Beclin 1/Mcl-1 negative co-regulation is dependent neither on transcriptional control nor on modulation of protein synthesis, suggesting that Mcl-1 and Beclin 1 mutually modulate the protein stability of each other. We next sought to examine the contribution of the lysosomal or proteasomal pathways to the degradation of Mcl-1 and Beclin 1. To this end, we treated 293T cells with specific pharmacological inhibitors of the two degradation processes. First, cells were treated at different time points in the presence or absence of either Bafilomycin A1 or a combination of E64d and pepstatin A, which are known to inhibit the lysosomal degradation pathway. As expected, both treatments led to the accumulation of LC3II confirming the impairment of lysosomal degradation, but no detectable changes were observed in either Mcl-1 or Beclin 1 protein levels ( Fig. 2e ). As opposed to lysosomal inhibition, proteasomal inhibition upon treatment with either MG132 or Epoxomicin led to an evident accumulation of Mcl-1 ( Fig. 2f ), as previously described [25] . In sharp contrast to the inverse correlation described earlier, increase in Mcl-1 protein level on inhibition of the proteasome was not associated with diminished Beclin 1 levels. Rather, Beclin 1 co-accumulated together with Mcl-1 ( Fig. 2f ), suggesting that the ubiquitin-proteasome pathway is the major turnover pathway for both Mcl-1 and Beclin 1. On the basis of this observation, we therefore explored the possibility that Mcl-1 and Beclin 1 can reciprocally modulate the proteasomal degradation of each other by affecting their ubiquitination. We assessed Beclin 1 ubiquitination status in 293T cells transfected with two independent siRNAs raised against Mcl-1. Knockdown of Mcl-1, as compared with control led to a significant reduction in the level of ubiquitinated Beclin 1. This effect was specific to Mcl-1 extinction, as siRNAs raised against other Bcl-2 family members, Bcl-2 or Bcl-xL, did not have any effect on the level of ubiquitinated Beclin-1 ( Fig. 2g ). Similarly, we also observed significant reduction in the level of ubiquitinated Mcl-1 when Beclin 1 was stably extinguished by two different shRNAs, as shown in Fig. 2h . Depletion of other regulators of autophagy Atg5 or Atg7 did not modulate Mcl-1 ubiquitination, further supporting the specificity of this regulation and its independency from autophagy. USP9X deubiquitinase interacts with both Mcl-1 and Beclin 1 As neither Mcl-1 nor Beclin 1 is known to exhibit direct ubiquitin ligase or deubiquitinase enzymatic activity, we investigated the possibility that Mcl-1 and Beclin 1 may indirectly regulate the ubiquitination of each other through modulating the binding or the function of other ubiquitination regulators (ubiquitin ligases or deubiquitinases). To systematically address this possibility, we profiled the entire interactomes of both Mcl-1 and Beclin 1 using mass spectrometry as an effective strategy for the identification of potential interacting ubiquitination regulators. Lysates from 293T cells transfected with expression vectors encoding Flag-tagged Mcl-1 or Beclin 1 were subjected to immunoprecipitation with an anti-Flag antibody. Interestingly, the mass spectrometric analysis of the co-immunoprecipitated proteins revealed that the USP9X deubiquitinase is a common interactor of both Mcl-1 and Beclin 1 ( Fig. 3a ). These results were then confirmed by immunoblotting analysis as shown in Fig. 3b , where USP9X is pulled down specifically only with Mcl-1 or Beclin 1, but not with Bcl-2 as a control. As a further control for specificity, we detected the presence of Mule, a known Mcl-1 interactor, only in the Mcl-1, but not the Beclin 1 immunoprecipitate. Furthermore, immunoprecipitation of endogenous USP9X showed that the interaction with Mcl-1 and Beclin 1 occurs at the level of endogenous proteins ( Fig. 3c ). Finally, immunofluorescence analysis showed an overlap in Mcl-1, Beclin 1 and USP9X localization ( Supplementary Fig. 3 ). 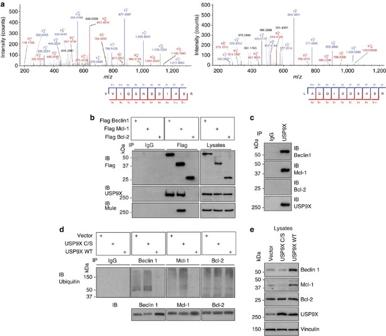Figure 3: USP9X binds, deubiquitinates and stabilizes Beclin 1 and Mcl-1. (a) Full annotation of two USP9X peptides identified by mass spectrometry in Beclin 1 or Mcl-1 complexes immunoprecipitated from 293T cells. (b) Biochemical validation of the interaction between USP9X and either Beclin 1 or Mcl-1 in 293T cells expressing the indicated constructs. (c) Physical binding between USP9X and both Beclin 1 and Mcl-1 at the endogenous protein levels in 293T cells. (d,e) Endogenous Beclin 1, Mcl-1 or Bcl-2 were immunoprecipitated from 293T cells transfected with constructs encoding USP9X WT or the enzymatically inactive USP9X C/S. The ubiquitination status of the immunoprecipitated proteins (d) as well as protein levels in total cell lysates (e) was assessed in each condition. Figure 3: USP9X binds, deubiquitinates and stabilizes Beclin 1 and Mcl-1. ( a ) Full annotation of two USP9X peptides identified by mass spectrometry in Beclin 1 or Mcl-1 complexes immunoprecipitated from 293T cells. ( b ) Biochemical validation of the interaction between USP9X and either Beclin 1 or Mcl-1 in 293T cells expressing the indicated constructs. ( c ) Physical binding between USP9X and both Beclin 1 and Mcl-1 at the endogenous protein levels in 293T cells. ( d , e ) Endogenous Beclin 1, Mcl-1 or Bcl-2 were immunoprecipitated from 293T cells transfected with constructs encoding USP9X WT or the enzymatically inactive USP9X C/S. The ubiquitination status of the immunoprecipitated proteins ( d ) as well as protein levels in total cell lysates ( e ) was assessed in each condition. Full size image USP9X deubiquitinates and stabilizes both Mcl-1 and Beclin 1 As USP9X has been previously shown to mediate Mcl-1 deubiquitination and stabilization [7] , we examined whether the interaction between USP9X and Beclin 1 has similar functional consequences. Endogenous Beclin 1, Mcl-1 or as a control Bcl-2 were immunoprecipitated from 293T cells transfected with constructs encoding wild type (WT) or enzymatically inactive mutant (C/S) USP9X. The ubiquitination status of the immunoprecipitated proteins was assessed by immunoblotting as described above. Overexpression of wild-type USP9X caused a significant reduction of the ubiquitination of Mcl-1, as expected, and of Beclin 1, which was not observed on overexpression of the USP9X catalytic mutant ( Fig. 3d ). USP9X overexpression, however, did not affect Bcl-2 to any extent. In line with these observations, wild-type USP9X overexpression but not the mutant USP9X C/S led to accumulation of both Mcl-1 and Beclin 1 as detected by immunoblotting analysis of total cell lysates ( Fig. 3e ). This effect seems to be specific to USP9X, as overexpression of another deubiquitinase, USP28, led to stabilization of its known substrate LSD1 but had no effect on Mcl-1 and Beclin 1 ubiquitination or total protein levels ( Supplementary Fig. 4a,b ). Mcl-1 and Beclin 1 compete for binding USP9X To get further insight into the role of USP9X in the regulation of Mcl-1 and Beclin 1, we next sought to map the binding regions of Mcl-1 and Beclin 1 on USP9X. To this end, different USP9X fragments ( Fig. 4a ) fused to GST and immobilized on glutathione beads were incubated with lysates of 293T cells expressing either Flag-tagged Beclin 1 or Flag-tagged Mcl-1. Beclin 1 and Mcl-1 bound the same USP9X fragment as shown in Fig. 4b . The fact that Mcl-1 is known to interact with both USP9X [7] and Beclin 1 [10] , [11] leaves open the possibility that USP9X could form a trimeric complex, rather than binding Beclin 1 and Mcl-1 individually. To investigate this possibility, we took advantage of obatoclax, a known inhibitor of the Bcl-2 family of protein that has been shown to disrupt the interaction between Mcl-1 and Beclin 1 (ref. 27 ). As shown in Fig. 4c , treatment of 293T cells with obatoclax, as expected, led to the disruption of the endogenous Beclin 1/Mcl-1 interaction. Under this condition, the binding of each individual protein to endogenous USP9X was not affected. These data indicate that Beclin 1 and Mcl-1 are able to bind endogenous USP9X independently of each other ( Fig. 4c ). 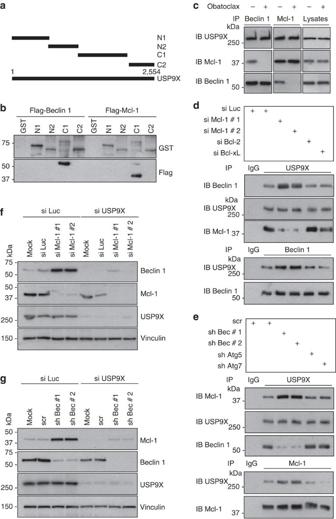Figure 4: Beclin-1 and Mcl-1 compete for USP9X binding. (a) Schematic representation of different USP9X fragments used for mapping the sites of interaction with Mcl-1 and Beclin 1 (b) GST-fused USP9X fragments were incubated with lysates from 293T cells expressing flag-tagged Beclin 1 or Mcl-1, and the interaction tested in pull-down assays. (c) Beclin 1/USP9X and Beclin 1/Mcl-1 interactions in 293T cells treated with or without Obatoclax. (d,e) Increase in USP9X/Beclin 1 and USP9X/Mcl-1 interactions on ablation of Mcl-1 or Beclin 1, respectively. USP9X, Beclin 1 or Mcl-1 were immunoprecipitated from 293T cells transfected with the indicated siRNAs/shRNAs. (f,g) USP9X is required for the reciprocal regulation between Mcl-1 and Beclin 1. Mcl-1 or Beclin 1 was knocked down in USP9X-depleted or control 293T cells, and the levels of the proteins were checked by immunoblotting. Figure 4: Beclin-1 and Mcl-1 compete for USP9X binding. ( a ) Schematic representation of different USP9X fragments used for mapping the sites of interaction with Mcl-1 and Beclin 1 ( b ) GST-fused USP9X fragments were incubated with lysates from 293T cells expressing flag-tagged Beclin 1 or Mcl-1, and the interaction tested in pull-down assays. ( c ) Beclin 1/USP9X and Beclin 1/Mcl-1 interactions in 293T cells treated with or without Obatoclax. ( d , e ) Increase in USP9X/Beclin 1 and USP9X/Mcl-1 interactions on ablation of Mcl-1 or Beclin 1, respectively. USP9X, Beclin 1 or Mcl-1 were immunoprecipitated from 293T cells transfected with the indicated siRNAs/shRNAs. ( f , g ) USP9X is required for the reciprocal regulation between Mcl-1 and Beclin 1. Mcl-1 or Beclin 1 was knocked down in USP9X-depleted or control 293T cells, and the levels of the proteins were checked by immunoblotting. Full size image Taken together, our data show that Mcl-1 and Beclin 1 reciprocally modulate the ubiquitination of each other with USP9X being a common interactor whose deubiquitinase activity stabilizes both of them, and that Mcl-1 and Beclin 1 independently bind the same region on USP9X. If the Beclin 1/Mcl-1 inverse co-regulation is a consequence of USP9X activity, one expectation would be that the relative level of Mcl-1 and Beclin 1 can influence the binding of each other to USP9X. To test this hypothesis, we examined the binding between USP9X and either Beclin 1 or Mcl-1 when the level of one of the latter two was diminished by RNAi. Depletion of Mcl-1, but not Bcl-2 or Bcl-xL as control, was associated with enhanced binding between Beclin 1 and USP9X ( Fig. 4d ). Similarly, enhanced binding between Mcl-1 and USP9X was detected in immunoprecipitates from 293T cells that have been depleted of Beclin 1, but not Atg 5 or Atg 7 ( Fig. 4e ). These results suggest a model in which both Mcl-1 and Beclin 1 compete with each other for binding USP9X. Decrease in the level of one relieves the competition for binding USP9X, which then impacts the ubiquitination and ultimately the protein level of the other. To further examine this model and to verify whether USP9X is indeed required for the reciprocal regulation of Beclin 1/Mcl-1 axis, we knocked down either Beclin 1 or Mcl-1 in control or USP9X-depleted cells. Stabilization of Mcl-1 or Beclin 1 in response to Beclin 1 or Mcl-1 knockdown, respectively, was greatly diminished in USP9X-depleted cells, confirming that USP9X mediates the reciprocal regulation between Mcl-1 and Beclin 1 ( Fig. 4f,g ). Our results further show that only a small fraction of USP9X is present in the membrane compartment in which most of the Mcl-1 and Beclin 1 localize, adding further significance to the competitive binding model ( Supplementary Fig. 5a,b ). Thus, these results suggest that the reciprocal regulation of ubiquitination and protein stability between Mcl-1 and Beclin 1 is associated with competitive displacement of USP9X. Beclin 1/Mcl-1 axis modulates melanoma growth Given the opposite roles of the two proteins in tumour cells, we sought to examine the implications of the identified reciprocal regulation of the Beclin 1/Mcl-1 axis in cancer and particularly explore whether the reported high levels of Mcl-1 and low levels of Beclin 1 in certain tumours are inter-dependent and could be explained by the identified mechanism of co-regulation. Expression of Beclin 1 is low in melanoma and the decrease in Beclin 1 levels was shown to correlate with melanoma progression [21] . Conversely, Mcl-1 has been associated with melanoma progression [28] and shown to be critical for survival of melanoma cells undergoing ER stress [29] or anoikis [30] . Mcl-1 has also been implicated in mediating resistance of melanoma cells to radiation [31] and several chemotherapeutic agents [32] , [33] , [34] . Using patient-derived melanoma as a relevant model of cancer, we first compared the levels of Mcl-1 and Beclin-1 proteins in a set of primary cultures of patient-derived melanoma cells and primary human melanocytes. Our data show that melanoma cells, as compared with melanocytes, express markedly lower levels of Beclin 1, which correlated with higher levels of Mcl-1. USP9X levels were comparable in both melanocytes and melanoma cells ( Fig. 5a ). 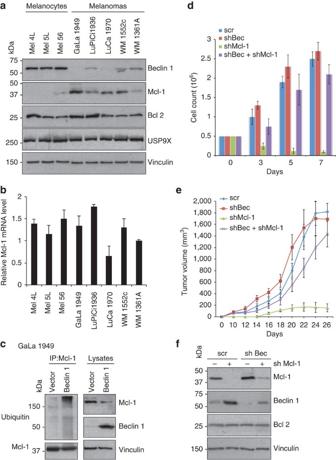Figure 5: Beclin 1/Mcl-1 axis modulates melanoma growthin vitroandin vivo. (a) Beclin 1 and Mcl-1 levels in patient-derived melanomas compared with primary melanocytes. (b) Mcl-1 mRNA levels in patient-derived melanomas and primary melanocytes. Error bars indicate s.e.m. (n=3 for all graphs). (c) Mcl-1 ubiquitination and degradation on transient expression of Beclin 1 in patient-derived 1949 melanoma cells. Endogenous Mcl-1 was pulled down from GaLa 1949 transiently transfected with Beclin 1 or empty vector and the level of Mcl-1 ubiquitination as well as total protein levels was assessed by immunoblotting. (d)In vitrogrowth of GaLa1949 melanoma cells expressing either scrambled shRNA or Beclin 1 shRNA upon ablation of Mcl-1 with doxycycline-inducible shRNA. Results are representative of at least three independent experiments. Error bars represent s.e.m. (n=3 for all graphs). (e)In vivogrowth of xenograft tumours derived from cells transduced with the indicated shRNA. Error bars indicate s.e.m. (n=8 per group). After establishment of xenografts, NSG mice were kept on 1 mg ml−1Dox supplemented in the drinking water to induce Mcl-1 shRNA. (f) Beclin 1 and Mcl-1 protein levels in xenografts isolated from animals in (c). Figure 5: Beclin 1/Mcl-1 axis modulates melanoma growth in vitro and in vivo . ( a ) Beclin 1 and Mcl-1 levels in patient-derived melanomas compared with primary melanocytes. ( b ) Mcl-1 mRNA levels in patient-derived melanomas and primary melanocytes. Error bars indicate s.e.m. ( n =3 for all graphs). ( c ) Mcl-1 ubiquitination and degradation on transient expression of Beclin 1 in patient-derived 1949 melanoma cells. Endogenous Mcl-1 was pulled down from GaLa 1949 transiently transfected with Beclin 1 or empty vector and the level of Mcl-1 ubiquitination as well as total protein levels was assessed by immunoblotting. ( d ) In vitro growth of GaLa1949 melanoma cells expressing either scrambled shRNA or Beclin 1 shRNA upon ablation of Mcl-1 with doxycycline-inducible shRNA. Results are representative of at least three independent experiments. Error bars represent s.e.m. ( n =3 for all graphs). ( e ) In vivo growth of xenograft tumours derived from cells transduced with the indicated shRNA. Error bars indicate s.e.m. ( n =8 per group). After establishment of xenografts, NSG mice were kept on 1 mg ml −1 Dox supplemented in the drinking water to induce Mcl-1 shRNA. ( f ) Beclin 1 and Mcl-1 protein levels in xenografts isolated from animals in ( c ). Full size image Consistent with a post-translational mode of upregulation, the elevated levels of Mcl-1 protein in melanoma cell lines did not correlate with higher Mcl-1 mRNA levels in comparison with melanocytes and did not generally correlate with the magnitude of Mcl-1 upregulation among different melanoma cell lines ( Fig. 5b ). Importantly, in patient-derived melanoma GaLa 1949 cells, forced expression of Beclin 1 led to enhanced Mcl-1 ubiquitination and decrease in Mcl-1 protein levels ( Fig. 5c ). Furthermore, proteasomal, but not lysosomal inhibition abolished the decline in Mcl-1 levels on Beclin 1 overexpression, indicating that Beclin 1-driven Mcl-1 degradation is mediated by the proteasome and is independent of autophagy ( Supplementary Fig. 6 ). Next, we investigated the relevance of Beclin 1/Mcl-1 axis to the tumorigenesis of melanoma. Melanoma cells were dependent on Mcl-1 upregulation for their proliferation as Mcl-1 knockdown in GaLa 1949 cells inhibited cell proliferation in vitro and impaired the growth of tumour xenografts in vivo ( Fig. 5d,e ). As in 293T and HeLa cells, Mcl-1 knockdown in GaLa cells was associated with an increase in Beclin 1 levels ( Fig. 5f ). This increase in Beclin 1 level was crucial for the observed block in proliferation upon Mcl-1 extinction, as cells depleted of both Mcl-1 and Beclin 1 proliferated almost normally in vitro and in vivo ( Fig. 5d,e ). The Beclin 1/Mcl-1 axis correlates with melanoma progression To further explore the observed role of the Beclin 1/Mcl-1 axis in melanoma, we next assessed Beclin 1 and Mcl-1 protein levels in lysates derived from either tumour-adjacent normal (N) or malignant (M) tissues of a set of melanoma patients. Immunoblotting analysis further confirmed the specific modulation of Beclin 1/Mcl-1 axis in human melanoma ( Fig. 6a ). Mcl-1 levels were consistently found higher in tumours as compared with normal tissues from the same patients. Conversely, in the same samples Beclin 1 protein levels were consistently found lower in tumour samples, inversely correlated with Mcl-1 levels. 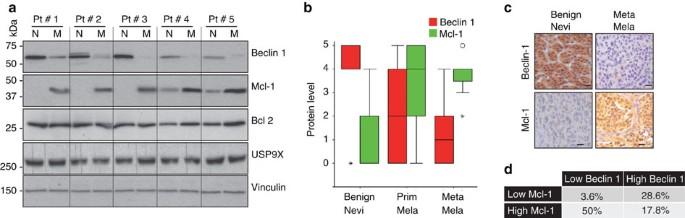Figure 6: Beclin 1/Mcl-1 axis contributes to the progression of melanoma. (a) Beclin 1 and Mcl-1 levels in lysates derived from either tumour-adjacent normal (N) or malignant (M) tissues of five melanoma patients. (b) Immunohistochemical analysis of Beclin 1 and Mcl-1 levels in patient samples of benign nevi (n=7), primary melanoma (Prim Mela,n=28) or metastatic melanoma (Meta Mela,n=8). The bars represent the highest and lowest quartiles. (c) Representative images of immunohistochemical analysis (original magnification, × 200) Scale bar, 40 μm. Figure 6: Beclin 1/Mcl-1 axis contributes to the progression of melanoma. ( a ) Beclin 1 and Mcl-1 levels in lysates derived from either tumour-adjacent normal (N) or malignant (M) tissues of five melanoma patients. ( b ) Immunohistochemical analysis of Beclin 1 and Mcl-1 levels in patient samples of benign nevi ( n =7), primary melanoma (Prim Mela, n =28) or metastatic melanoma (Meta Mela, n =8). The bars represent the highest and lowest quartiles. ( c ) Representative images of immunohistochemical analysis (original magnification, × 200) Scale bar, 40 μm. Full size image Moreover, immunohistochemical staining of patient-derived benign nevi, primary melanoma or metastatic melanoma revealed a highly significant negative rank correlation between Mcl-1 and Beclin 1 levels (Sperman’s rho=−0.713, N =43; P =0.000001) ( Fig. 6b,c ). Mcl-1 tended to increase and Beclin 1 decreased as lesions progressed to a more malignant phenotype (χ 2 =11.93; n =2; P =0.003** and χ 2 =8.09; n =2; P =0.018* at Kruskal Wallis Test, respectively) ( Fig. 6b,c ). Even within the more heterogeneous population of primary melanoma, the inverse rank correlation between Mcl-1 and Beclin 1 levels was statistically significant (Sperman’s rho=−0.580; N =28; P =0.001). While most of the primary melanoma samples expressed low Beclin 1 levels and corresponding high levels of Mcl-1, in the majority of primary melanoma samples that expressed high level of Beclin 1, Mcl-1 level was low further confirming their inter-dependency ( Fig. 6d ). Moreover, Mcl-1 and Beclin 1 levels showed a slight trend towards a respectively negative and positive correlation with survival of patients (Spearman’s rho=−0.259; N =35; P =0.133 and rho=0.223; N =35; P =0.198, respectively). Taken together, these data confirm that in melanoma as a relevant cancer model, the levels of Mcl-1 and Beclin 1 proteins are inversely co-regulated as observed in other cell models. Importantly, our results show that the Beclin 1/Mcl-1 axis is specifically modulated during melanoma progression with Beclin 1 level decreasing and Mcl-1 increasing in a statistically significant correlation, strongly suggesting that the change in the level of the two proteins is closely interdependent. Here we unravel a novel regulatory mechanism that not only is essential for the regulation of Mcl-1 but also reciprocally regulates the haplo-insufficient tumour suppressor Beclin 1. In several cell models, modulation of either Beclin 1 or Mcl-1 level impacted the protein level of the other in an inverse manner. Beclin 1 plays an essential role in the process of autophagy. However, the modulation of Mcl-1 by Beclin 1 seems to be independent of autophagy as depletion of other autophagy proteins Atg 5 and Atg 7 did not lead to changes in Mcl-1 levels and in contrast to proteasomal inhibition, lysosomal inhibition did not modulate the decline in Mcl-1 level on Beclin 1 overexpression. This effect is also independent of the physical interaction between Beclin 1 and Mcl-1. We demonstrate that the inverse reciprocal regulation between Beclin 1 and Mcl-1 is mediated by competitive binding to the common deubiquitinase USP9X, which consequently determines their ubiqitination and proteasomal degradation. Mcl-1 is upregulated in several types of cancer. Melanoma is an example of tumours in which Mcl-1 plays crucial tumour-promoting roles by promoting survival on anoikis [30] and endoplasmic reticulum stress [29] and mediating resistance to radiation [31] and several anticancer agents such as Fas [32] , dacarbazine [33] and ABT737 (ref. 34 ). Moreover, in the light of our results and the recent reports that implicate Mcl-1 in the regulation of autophagy, mitochondrial respiration and ATP production [8] , [10] , [11] , Mcl-1 may contribute to the survival and progression of melanoma not only by evading apoptosis but also by affecting tumour cell energetics. Several pathways are implicated in the regulation of Mcl-1 expression, translation and degradation. However, the contribution of these pathways to the observed upregulation of Mcl-1 in different types of tumours is not clear. In T-cell acute lymphoblastic leukaemia, follicular lymphoma, small cell lung carcinomas, ductal and colon adenocarcinoma, high Mcl-1 levels have mainly been attributed to decreased proteasomal degradation and increased stability of Mcl-1 protein [7] , [35] . Using patient-derived melanoma cells and tissue samples of benign and malignant melanocytic lesions at different stages, we show that melanomas express low levels of Beclin 1 and closely corresponding high levels of Mcl-1. Our data thus establish a significant inverse correlation between Beclin 1 downregulation and elevated Mcl-1 levels in melanoma. Importantly, forced expression of Beclin 1 in patient-derived melanoma cells reduced Mcl-1 levels and knockdown of either Mcl-1 or Beclin 1 showed that the modulation of the level of one of the two inversely impacts levels of the other, clearly confirming the interdependency of the changes in levels of the two proteins in melanomas models as sketched in Fig. 7a . Our results also show that changes in Beclin 1/Mcl-1 axis modulate the proliferation of melanoma cells and correlate with melanoma progression ( Fig. 7b ). 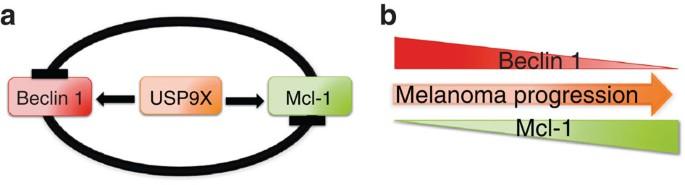Figure 7: Model of Beclin 1/Mcl-1 co-regulation and contribution to melanoma progression. Schematic representation of competitive binding of Mcl-1 and Beclin 1 to USP9X (a) and the correlation between Beclin 1/Mcl-1 axis and melanoma progression (b). Figure 7: Model of Beclin 1/Mcl-1 co-regulation and contribution to melanoma progression. Schematic representation of competitive binding of Mcl-1 and Beclin 1 to USP9X ( a ) and the correlation between Beclin 1/Mcl-1 axis and melanoma progression ( b ). Full size image Interestingly, while Beclin 1 and Mcl-1 showed a general trend to decrease and increase, respectively, with the progression of melanocytic lesion from benign nevi to metastatic melanoma, in the samples of primary melanoma with relatively higher level of Beclin 1, the level of Mcl-1 was accordingly lower and vice versa. The inverse rank correlation between Mcl-1 and Beclin 1 levels within this heterogeneous population was statistically significant further confirming the interdependency of the levels of both proteins. The tight inverse correlation and marked changes in Mcl-1 and Beclin 1 protein levels in correspondence to each other suggest that this mechanism of co-regulation is a major determinant of the Beclin 1/Mcl-1 axis. The mechanisms by which Beclin 1 suppresses tumorigenesis remain largely unravelled but generally assumed to be linked to its essential role in the regulation of autophagy. However, it is not clear whether autophagy solely accounts for Beclin 1 tumour suppressive capacity. First, autophagy plays controversial or possibly dual role in cancer. Second, Beclin 1 is unique among other autophagy-regulating genes in several ways: unlike most other autophagy-regulating genes such as Atg3, Atg4C, Atg5, Atg7, Atg9, Atg16L1 and ULK , BECN1 knockout in mice is embryonically lethal. Furthermore, in contrast to BECN1 hemizygous animals, Atg5 and Atg7 hemizygous mice do not develop spontaneous tumours [36] . It is thus likely that Beclin 1 plays autophagy-independent roles in other processes that may contribute to its tumour-restraining potential. Indeed, multifunctional role of Beclin 1 in cellular processes is now emerging [22] , [23] . The ability of Beclin 1 to modulate Mcl-1 level according to the mechanism we unravel in this study could thus be an autophagy-independent function of Beclin 1 that contributes to its tumour suppression capacity. From another angle, mutations that lead to increased Mcl-1 levels may contribute to tumorigenesis by destabilizing Beclin 1 and thus evading its tumour suppression actions. With the ability of USP9X to stabilize both the tumour-promoter Mcl-1 as well as the tumour suppressor Beclin 1, the net contribution of USP9X to tumorigenesis is probably more complex than initially thought. Indeed, recent reports suggest both tumour promoting as well as tumour suppressive functions for USP9X in different contexts [7] , [37] . It will be relevant in the future to identify the factors that dictate the positive or negative contribution of USP9X to tumorigenesis, and govern its substrate specificity and recruitment, and to study how its cellular distribution may regulate its availability for interacting proteins. Reagents The following antibodies were used at working dilution of 1:1,000, unless otherwise mentioned: anti-LC3 (MPL Biomedicals); anti-p62, anti-Beclin-1 and anti-Mcl-1 (Santa Cruz Biotechnology); anti-Bcl-2 and anti-Bcl-xL (BD Biosciences); anti-Noxa (Calbiochem); anti-Beclin-1, anti-Atg5, (Novus) and anti-Atg7 (Epitomics); anti-FLAG (M2-SIGMA, dilution 1:2,000); anti-Vinculin (h-VIN1, SIGMA, dilution 1:1,0000); anti-Bad (Cell Signaling Technology); anti-Mule and anti-USP9X (Bethyl Laboratories). Doxycycline, Cycloheximide, E64d, pepstatin A, Bafilomycin A1 and Epoxomicin were purchased from Sigma Aldrich. Sorafenib, Roscovitine, ABT737 and MG132 were purchased from Selleck Chemicals. Flag-tagged Mcl-1 was obtained from addgene.org, Flag-tagged Beclin 1 was kindly provided by Dr Beth Levine and USP9X constructs were kindly provided by Dr Simona Polo. Tissue culture HEK293T cells were acquired from the American Type Culture Collection (ATCC, Manassas, VA) and were grown in Dulbecco’s modified Eagle’s medium supplemented with 10% fetal bovine serum and 2 mM L -glutamine. HeLa cells and patient-derived melanoma cells were grown in RPMI supplemented with 10% fetal bovine serum and 2 mM L -glutamine. Primary human melanocytes Mel 4L, Mel 5L and Mel 56 were isolated from surgical dissection according to the standardized protocols. Biological samples for research purposes were collected from patients whose informed consent was obtained in writing according to the policies of the Ethics Committee of the European Institute of Oncology and regulations of Italian Ministry of Health. Cells were cultured in McCoy’s 5A Medium (Invitrogen) supplemented with: 2% FBS, 5 μg ml −1 recombinant human Insulin, 5 μg ml −1 human Transferrin, 0.5 μg ml −1 Hydrocortisone, 20 pm Cholera Toxin from Vibrio cholerae, 16 nm Phorbol 12-myristate 13-acetate, 10 nm human Endothelin 1, 10 ng ml −1 recombinant human SCF and 1 ng ml −1 recombinant human FGF-2. All cultures were maintained in a humidified tissue culture incubator at 37 °C in 5% CO 2 . Establishment of primary cultures from metastatic melanomas Tumour specimens (at least 1 g) were put in Petri dishes containing RPMI 1640+10% FCS. After eliminating non-tumour and necrotic parts, tissue was dissected into small pieces with a scalpel, squeezing each piece for allowing cells to go into suspension. Cell suspension was filtered through sterile gauze to eliminate macroscopic debris. Cell suspension was checked for cellular composition: in the presence of significant red blood cell contamination, treatment with ACK (10 min on ice) was performed, the samples were centrifuged and dead cells eliminated by digestion with DNase and trypsin treatment. Viability of cell suspension was checked by trypan blue exclusion. In the case when the number of tumour cells obtained from the mechanical processing was not adequate, the remaining tumour tissue fragments were treated with a series of enzymes: DNase (200 UI ml −1 ), collagenase (0.1%), hyaluronidase (2.5 UI ml −1 ) and Trypsin (0.5 mg ml −1 ). Following 45-minute incubation at room temperature on a magnetic shaker, cell suspension was filtered through sterile gauze to remove debris. Cell suspension was recovered from the supernatant by centrifugation and extensively washed in RPMI 1640+10% FCS. Cells were grown in DMEM+10% FBS and were periodically characterized by immunohystochemistry staining with S100, MelanA and HMB45 antibodies at various passages during the time they are kept in culture. RNA interference siRNA oligos were purchased from Dharmacon. shRNA pLKO.1 lentiviral constructs were purchased from Open Biosystems. Doxycycline-inducible shMcl-1 construct was obtained by cloning shMcl-1 sequence # 1 in pLKO-Tet-On lentiviral vector (Open Biosystems). Target sequences are mentioned in Supplementary Table 1 . Transfection of mammalian cells 293T cells were transiently transfected using Lipofectamine 2000 reagent (Invitrogen) according to the manufacturer’s protocol. In brief, Lipofectamine 2000 was added to OptiMEM (Invitrogen). Lipofectamine 2000-OptiMEM mix was added dropwise to the plasmid/siRNAs and was allowed to settle for 15 min before it was added to cells. GaLa 1949 cells were electroporated using Amaxa Nucleofection procedures. In brief, cells were trypsinized, pelleted and resuspended in nuclefection buffer. Hundred microlitres of the cell suspension was added to plasmid mix, transferred to a nucleofection cuvette and immediately nucleofected using Amaxa nucleofector. Five hundred microlitres of fresh medium was added immediately to the cells after nucleofection and the nucleofection mix was seeded in a 10-cm dish containing 8 ml of pre-warmed medium. Lentiviral transduction The pLKO.1 vectors and package plasmids were co-transfected into packaging HEK293T cells, and the viral supernatants were collected and used to infect target cells in four 2-h cycles of transduction over two consecutive days. Immunoblotting Total cell lysates were prepared by lysing cells or cell pellets in SDS–PAGE lysis buffer (100 mM Tris.HCl pH6.8, 4%SDS, 20% glycerol, 0.1% bromophenol blue and 5% β-mercaptoethanol added immediately before use) followed by heating at 94 °C for 7 min. Lysates were then electrophoresed on 8–15% SDS–PAGE gels. Gels were run at 100 V (stacking gel)/150 V (separation gel) on Protean III apparatus (BioRad). Gels were transferred onto nitrocellulose and probed with the appropriate primary antibody for a variable incubation time depending on the experimental design, followed by the corresponding secondary antibodies diluted 1:1,000. The proteins were visualized by enhanced chemiluminescence (ECL), according to the manufacturer’s instructions (Amersham Pharmacia Biotech). Representative uncropped scans of blots generated with the most relevant antibodies used along the different figures are presented in Supplementary Fig. 7 . Immunoprecipitation Cells were lysed in IP lysis buffer (150 mM NaCl, 50 mM HEPES, pH 7.5, 1% triton X100, 1 mM EDTA and 10% glycerol) freshly supplemented with 1 mM DTT, protease inhibitor cocktail (Roche), phosphatase inhibitor cocktail, 1 mM N-ethylmaleimide (NEM). Cell lysates were pre-cleared by incubation for 2 h at 4 °C with pre-immune serum. Supernatants were then incubated for 4 h with the indicated antibodies at working dilution of 1:100 or control IgG under constant rotation at 4 °C. Beads were washed five times in ice cold lysis buffer containing 0.1%Triton X100. Beads were finally collected by centrifugation at 5,000 g for 2 min and brought up in SDS-PAGE lysis buffer for further analysis. For in vivo GST pull-down assay, lysates of 293T cells expressing Flag Beclin 1 or Flag-Mcl-1 were incubated with GST or GST-fused proteins and 20 μl of glutathione-Sepharose 4B at 4 °C under constant rotation for 2 h and washed four times with washing buffer (20 mm Tris-HCl, pH 7.4, 150 mm NaCl, 0.1% SDS, 1 mm EDTA). Mass spectrometry Proteins were extracted in SDS-PAGE sample buffer and separated by one-dimensional electrophoresis using a 4–12% polyacrylamide Nu-PAGE Novex Bis-tris gel (Life Technologies, Paisley, UK). Peptides were analysed by RP-chromatography on an Agilent 1100 LC system (Agilent Technologies) coupled to LTQ-FT ultra (Thermo Fisher Scientific). MS data were analysed for protein identification using Mascot Daemon v.2.3.2 set up with the following parameters: Database Swiss prot; Taxonomy Homo Sapiens; Enzyme trypsin; Max missing cleavage 2; Fixed mod carbamidomethyl (C); Variable mod oxidation (M); Peptide tolerance 10 p.p.m. ; MS/MS tolerance, 0.5 Da; Instrument, ESI-TRAP. Cellular fractionation 293T and GaLa1949 cells were fractionated using the Qproteome Cell Compartment Kit (Qiagen) according to manufacturer’s protocol. Immunofluorescence 293T cells plated on cover slips were permeabilized using 0.2% Triton X100 (in 10% glucose, 25 mM PIPES pH 6.8, 1 mM EGTA and 1 mM MgCl2) for 5 min at room temperature to extract most of the soluable cytosolic proteins and fixed with 4% paraformaldehyde for 10 min at room temperature. Cells were then washed twice with PBS (pH 7.2) and blocked for 30 min with 2% BSA and then for 1 h at room temperature with fluorochrome-conjugated antibodies diluted 1:100 in blocking buffer, washed three times with PBS. Finally, cells were stained with DAPI for 5 min, mounted with glycerol and examined with Leica TCS SP2 AOBS confocal microscope with a × 60 objective under oil immersion. Xenografts NOD scid gamma (NSG) mice ( n =8 per group) received single subcutaneous flank injections of 1 × 10 6 patient-derived melanoma cells transduced with different shRNAs and diluted in 200 μl saline. Seven days later, mice were given drinking water containing 1 mg ml −1 doxycycline and 1% sucrose for induction of Mcl-1 shRNA expression in vivo . Tumour growth was monitored by bidimensional measurements using a calliper. Experiments have been done in accordance with the Italian Laws (D.L.vo 116/92 and following additions), which enforces EU 86/609 Directive (Council Directive 86/609/EEC of 24 November 1986 on the approximation of laws, regulations and administrative provisions of the Member States regarding the protection of animals used for experimental and other scientific purposes). Mice have been housed accordingly to the guidelines set out in Commision Recommendation 2007/526/EC 18 June, 2007 on guidelines for the accommodation and care of animals used for experimental and other scientific purposes (project number 02/12). Immunohistochemistry Immunohistochemical staining was performed on 3- μ m-thick sections of the most representative tumour paraffin block, using the streptavidin-biotin method. Sections were dewaxed, pretreated in a bath (Lab Vision PT Module) (Bio-Optica, Milan, Italy), with WCAP citrate buffer, pH 6.0 (Bio-Optica), for 40 min at 98.5 °C, and incubated with 3% H2O2 in TBS to inhibit endogenous peroxidase. The primary antibodies were then applied at working dilution of 1:50. To improve the immuno-reactivity of antigens, we used the UltraVision LP Large Volume Detection System HRP or AP Polymer (Ready-To-Use) (Bio-Optica), with either diaminobenzidine (Dako, Milan, Italy) for 8 min or new fuchsin for 7 min (Bio-Optica), as chromogens, respectively. All sections were then counterstained with Meyer’s haematoxylin. For each antibody, negative controls were obtained by replacing the primary antibody with a non-immune serum at the same concentration. Immunostaining was semi-quantitatively evaluated based on both the percentage of positive tumour cells (0, ≤10%; 1, >10% and ≤50%; 2, >50%) and the intensity of stain (0, absent; 1, weak; 2, moderate; 3, strong). Score ranged from 0 to 5 (4 and 5 were considered high scores). How to cite this article: Elgendy, M. et al. Beclin 1 restrains tumorigenesis through Mcl-1 destabilization in an autophagy-independent reciprocal manner. Nat. Commun. 5:5637 doi: 10.1038/ncomms6637 (2014).